Ultrasonic frogs show extraordinary sex differences in auditory frequency sensitivity Acoustic communication has an important role in the reproductive behaviour of anurans. Although males of the concave-eared frog ( Odorrana tormota ) have shown an ultrasonic communication capacity adapted to the intense, predominately low-frequency ambient noise from local streams, whether the females communicate with ultrasound remains unclear. Here we present evidence that females exhibit no ultrasonic sensitivity. Acoustic playback experiments show that the calls from male evoke phonotaxis and vocal responses from gravid females, whereas the ultrasonic components (frequencies above 20 kHz) of the calls do not elicit any phonotaxis or vocalization in the females. Electrophysiological recordings from the auditory midbrain reveal an upper frequency limit at 16 kHz in females. Laser Doppler vibrometer measurements show that the velocity amplitude of the tympanic membranes peaks at 5 kHz in females and at ∼ 7 kHz in males. The auditory sex differences in O. tormota imply that ultrasonic hearing has evolved only in male anurans. Acoustic communication has an important role in the reproductive behaviour of anurans. The Chinese concave-eared frog Odorrana tormota is an arboreal, nocturnal species that lives in the Huangshan Mountains, China amidst streams, which produce low-frequency ambient noise. During the reproductive season, males emit a variety of high-pitched calls (for example, long call, short call and staccato call) at night with energy spectrums extending into the ultrasonic range [1] , [2] , [3] , [4] . Gravid females produce courtship calls that are distinct from the males' advertisement calls, having higher fundamental frequencies, multiple harmonics and shorter call duration [2] . Furthermore, female calls evoke vocalizations and precise positive phonotaxis in males. Thus, O. tormota is the first non-mammalian vertebrate shown to communicate with ultrasonic frequencies ( ≧ 20 kHz), and male frogs' sunken tympana are hypothesized to have a key role in their high-frequency hearing sensitivity. However, females, unlike males, have thicker eardrums and no ear canals and whether they detect ultrasound is unclear. To understand the male–female interaction, we performed indoor playback experiments close to their natural habitat of the male's call to the female. We found that female frogs respond with positive phonotaxis and vocalizations to broadcasts of conspecific male calls, but not to the ultrasonic components of the calls. The behavioural study was complemented by electrophysiological recordings from the auditory midbrain and by laser Doppler vibrometer measurements of tympanic membrane's (TM) response to acoustic stimuli. These data demonstrate that there are noticeable sex differences in hearing between the sexes of O. tormota . Playback experiments After gravid female frogs were captured at night from their natural habitat, we immediately carried out acoustic playback experiments in a quiet and darkened room, where an area (150 cm length×90 cm width) was padded with acoustic foams. The three basic call-types of the male's vocalizations (long call, short call and staccato call) [2] , [4] and their filtered ultrasonic components (frequency ≧ 20 kHz) were used as acoustic stimuli and played back through the Play unit, a loudspeaker (pass band 0.1–40 kHz) and an ultrasonic loudspeaker (pass band 22–120 kHz) at a rate of one stimulus per 15 s, 90 dB SPL (sound pressure level) [2] , [5] . The playbacks of long or short calls frequently evoked movement (for example, jump and/or creep) in the gravid females. A female oriented her body towards the loudspeakers and then hopped onto the speakers with one or more jumps per trial (jump range: ~40–100 cm) with a localization error of 1.3±1.7 o (mean±s.d., 60 jumps, n =12 females; Fig. 1a ) under the long call (53 of 60, 88.3%; Supplementary Movies 1 and 2 ), short call (4 of 60, 6.7%; Supplementary Movie 3 ) and staccato call stimulation (3 of 60, 5%). When staccato call stimuli (a dominant frequency of ∼ 4 kHz) were presented, gravid females crept rapidly to the loudspeakers with a latency of 4.2±3.0 s (mean±s.d., n =6). 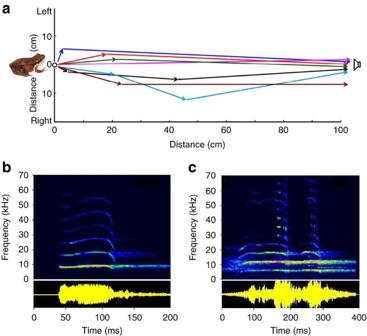Figure 1: Phonotactic movements and vocal responses in femaleO. tormotaelicited by playback of the male calls. (a) Representative phonotactic responses of gravid females in an area (150 cm length×90 cm width), showing long-distance jumps (range: 40–100 cm) with an average localization error of 1.3±1.7° (mean±s.d.; 60 jumps,n=12 females) towards the loudspeakers broadcasting the male's long call. Arrows denote the direction and extent of each jump. The inset is a picture of a gravid female frog. (bandc) Spectrogram (above) and waveform (below) of an evoked vocal response (EVR) from a gravid female frog (b) elicited by the male's long-call stimulus (c) with latency of 6.5 s. The EVR consists of a frequency-modulation pip with multiple harmonics having the fundamental frequency (F0) of 7.9–9.3 kHz (b), higher than theF0(∼6.0 kHz) of the long-call stimulus (c). Figure 1: Phonotactic movements and vocal responses in female O. tormota elicited by playback of the male calls. ( a ) Representative phonotactic responses of gravid females in an area (150 cm length×90 cm width), showing long-distance jumps (range: 40–100 cm) with an average localization error of 1.3±1.7° (mean±s.d. ; 60 jumps, n =12 females) towards the loudspeakers broadcasting the male's long call. Arrows denote the direction and extent of each jump. The inset is a picture of a gravid female frog. ( b and c ) Spectrogram (above) and waveform (below) of an evoked vocal response (EVR) from a gravid female frog ( b ) elicited by the male's long-call stimulus ( c ) with latency of 6.5 s. The EVR consists of a frequency-modulation pip with multiple harmonics having the fundamental frequency ( F 0 ) of 7.9–9.3 kHz ( b ), higher than the F 0 ( ∼ 6.0 kHz) of the long-call stimulus ( c ). Full size image In particular, the playback of the male long call, short call or staccato call elicited an evoked vocal responses (EVRs) from the gravid females, beginning immediately after the stimulus onset (delay time, mean±s.d., 7.16±2.43 s; 34 EVRs, n =8; Supplementary Movies 4 and 5 ). The female's evoked vocalizations are characteristic of a frequency-modulation pip with multiple harmonics ( Fig. 1b ) and have an F 0 of 8.13±0.97 kHz ( n =8), which is higher than the F 0 of the male long call ( ∼ 6.0 kHz; Fig. 1c ). The EVR is probably important for mate location, because female courtship calls can in turn induce receptive males' antiphonal calls, and rapid and hyperacute phonotactic approaches, as demonstrated in a previous study [2] . All actions facilitate successful mating amidst low-frequency ambient noise produced by nearby streams and waterfalls. However, neither EVR nor movement could be evoked from the examined 12 females by playbacks of filtered ultrasonic components of the male calls. This indicates that females of O . tormota are insensitive to ultrasound, and the ultrasound components of the calls therefore function in male–male territorial interactions [1] , [2] . Electrophysiological experiments To physiologically validate the behavioural observation of female O . tormota having no ultrasonic sensitivity, extracellular auditory evoked potential (AEP) from the torus semicircularis (TS; the frog's auditory midbrain) was recorded indoors in response to tone bursts (frequency range 1–35 kHz). The female AEPs were consistently observed in response to tone bursts at frequencies between 1 and 14 kHz, at a constant intensity of 90 dB SPL, and occasionally at 15 kHz, 103 dB SPL ( Fig. 2a ). No AEP was detected from 17 females using stimuli at frequencies above 16 kHz and at an intensity of 110 dB SPL. 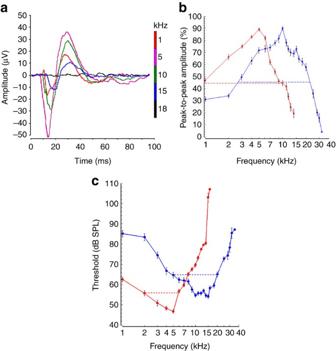Figure 2: Averaged auditory-evoked potential data from the torus semicircularis ofO. tormota. (a) Representative AEP waveforms recorded from the female TS in response to 20 tone bursts presented at frequency range 1–14 kHz, a rate of 1 s−1and 90 dB SPL. The AEP (blue curve) was recorded at 15 kHz, 103 dB SPL; AEP (black curve) at 18 kHz, 110 dB SPL. (b) Normalized peak-to-peak amplitudes of the AEPs as a function of tone frequency. Independent samples two-tailedt-test:t5 kHz=5.93,P<0.0001;t10 kHz=11.49,P<0.0001 (n=17 females, red curve;n=22 males, blue curve). The frequency widths at half maximum are illustrated for males and females respectively (dashed line). (c) Averaged AEP thresholds versus frequency relationships. Independent samples two-tailedt-test:t5 kHz=8.54,P<0.0001;t10 kHz=9.35,P<0.0001 (n=17 females, red curve;n=22 males, blue curve). Dashed lines indicate the auditory-sensitive frequency bandwidth (at 10 dB above threshold at characteristic frequency, CF). Error bars are ±1 s.e.m. The peak-to-peak AEP amplitudes measured at 90 dB SPL were normalized and plotted with a log-frequency axis in Figure 2b (mean±s.e.m. ; 95 AEP's, n =17 females; 61 AEP's, n =22 males), which showed significant sex differences in the mean amplitude with a single prominent peak at 5 kHz in females (red curve) versus 10 kHz in males (blue curve; independent samples two-tailed t -test: t 5 kHz =5.93, P <0.0001; t 10 kHz =11.49, P <0.0001; n , 17 females, 22 males). The frequency width at half maximum of the averaged AEP amplitude compared with frequency curves (dashed line) ranged from ∼ 3 to 22 kHz for males versus from ∼ 1 to 10 kHz for females. Figure 2: Averaged auditory-evoked potential data from the torus semicircularis of O. tormota . ( a ) Representative AEP waveforms recorded from the female TS in response to 20 tone bursts presented at frequency range 1–14 kHz, a rate of 1 s −1 and 90 dB SPL. The AEP (blue curve) was recorded at 15 kHz, 103 dB SPL; AEP (black curve) at 18 kHz, 110 dB SPL. ( b ) Normalized peak-to-peak amplitudes of the AEPs as a function of tone frequency. Independent samples two-tailed t -test: t 5 kHz =5.93, P <0.0001; t 10 kHz =11.49, P <0.0001 ( n =17 females, red curve; n =22 males, blue curve). The frequency widths at half maximum are illustrated for males and females respectively (dashed line). ( c ) Averaged AEP thresholds versus frequency relationships. Independent samples two-tailed t -test: t 5 kHz =8.54, P <0.0001; t 10 kHz =9.35, P <0.0001 ( n =17 females, red curve; n =22 males, blue curve). Dashed lines indicate the auditory-sensitive frequency bandwidth (at 10 dB above threshold at characteristic frequency, CF). Error bars are ±1 s.e.m. Full size image Figure 2c delineates the averaged thresholds versus frequency relationships in the females and males of O. tormota , respectively, showing the characteristic frequency (CF), or frequency of minimum threshold, at 5 kHz in females (mean±s.e.m. ; 46.9±0.9 dB SPL; n =17 females; red curve), and at 10 kHz (54.8±0.87 dB SPL; n =22 males) and 15 kHz in males (54.1±0.84 dB SPL; n =22 males; blue curve). There are significant differences in the mean thresholds at 5 and 10 kHz between males and females, respectively (independent samples two-tailed t -test: t 5 kHz =8.54, P <0.0001; t 10 kHz =9.35, P <0.0001; n , 17 females, 22 males). The audible upper frequency limit was found at 16 kHz (107 dB SPL) in females and at 35 kHz (87 dB SPL) in males. Moreover, the auditory sensitive frequency bandwidth (at 10 dB above threshold at CF) ranged from 2 to 6 kHz in females and from 5 to 20 kHz in males ( Fig. 2c ; dashed line). The male frog is ∼ 10 dB less sensitive than the female. The Q 10 (CF/bandwidth at 10 dB above threshold) of the averaged thresholds versus frequency relationships were calculated for females (mean±s.d. ; 1.42±0.68, n =17) and for males (0.93±0.31, n =22), indicating that the differences in the sharpness of frequency tuning (Q 10 ) in males and females are significantly different (independent samples two-tailed t -test: t =3.00, P <0.01; n , 17 females, 22 males). A total of 218 single units were recorded from the TS of the species (108 units from 11 females and 110 units from 30 males) to determine the best excitatory frequency (BEF) at the lowest intensity. The distribution of single units' BEFs in females notably differed from that in males, as shown in the histogram ( Fig. 3a ) and line chart ( Fig. 3b ). For females, most units (82.4%, 89/108 units) had BEF between 4 and 6 kHz with a peak at 5 kHz (38.9%, 42/108), and no unit of BEF >10 kHz was found, whereas in males approximate half the units (44.5%, 49/110) had BEF between 8 and 10 kHz, 16.4% (18/110) between 14 and 16 kHz, and 2.7% (3/110) at 20 kHz. There is a substantial difference in the distributions of the TS units' BEF between both sexes ( F -test: F =3.73 >2.12 ( F 19,19 ), P =0.003). The line chart is characterized by both the kurtosis (ku) and skewness (sk) of the two data sets. The measurements reveal that the BEF data set in females with high kurtosis (ku f =5.73) tends to have a distinct peak near 5 kHz, which declines rapidly, and the distribution is unimodal. In contrast, the BEF data set in males, with a much lower kurtosis (ku m =0.44), tends to have a flat top near the frequency range of 8–10 kHz rather than a sharp peak, and the continuous distribution has multiple different modes, which appear as distinct peaks (local maxima). In addition, the skewness in females (sk f =2.45) was higher than that in males (sk m =1.18). For the females, the tapering tail on the right side is longer than the left side of the figure, which indicates that the mass of the distribution is concentrated on the left, whereas in males the values are distributed on both sides of the frequency range of 8–10 kHz. Thus, electrophysiological data demonstrate that sex differences in the auditory frequency filters observed in the concave-eared frog O . tormota are notable in comparison with previous studies on three species of frogs: Elentherodactylus coqui [6] , Acris crepitans [7] and Hyla ebraccata [8] . 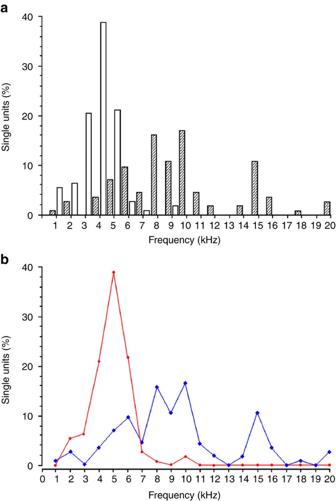Figure 3: Single-unit best excitatory frequency data from the torus semicircularis ofO. tormota. (a) Histogram of the BEF of 218 TS units (108 units,n=11 females, open bar; 110 units,n=30 males, hatching bar), showing the number of single units (%) at different frequency (kHz). There is substantial difference in the BEF distribution of TS units between females and males (F-test:F=3.73 >2.12 (F19,19),P=0.003). (b) Line chart of the BEF of 218 units (108 units,n=11 females, red line; 110 units,n=30 males, blue line), showing the distribution of the number of single units (%) at different frequency (kHz). Both the kurtosis (ku) and skewness (sk) are measured: kuf=5.73, skf=2.45 in females; kum=0.44, skm=1.18 in males. Figure 3: Single-unit best excitatory frequency data from the torus semicircularis of O. tormota . ( a ) Histogram of the BEF of 218 TS units (108 units, n =11 females, open bar; 110 units, n =30 males, hatching bar), showing the number of single units (%) at different frequency (kHz). There is substantial difference in the BEF distribution of TS units between females and males ( F -test: F= 3.73 >2.12 ( F 19,19 ), P =0.003). ( b ) Line chart of the BEF of 218 units (108 units, n =11 females, red line; 110 units, n =30 males, blue line), showing the distribution of the number of single units (%) at different frequency (kHz). Both the kurtosis (ku) and skewness (sk) are measured: ku f =5.73, sk f =2.45 in females; ku m =0.44, sk m =1.18 in males. 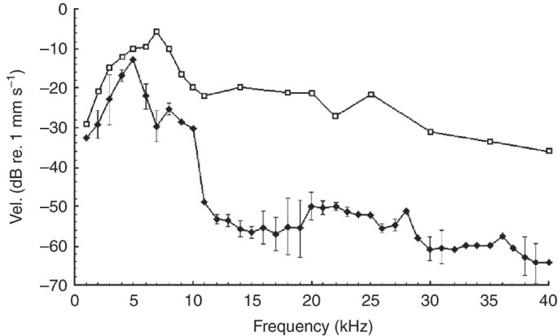Figure 4: Vibration velocity amplitude of the tympanic membrane ofO. tormotain response to sound. Velocity amplitude spectrum of the female's TM (solid diamonds), showing a peak around 5 kHz. Measurements at frequency range 1–40 kHz and 80 dB sound pressure level were made from five eardrums of three females. The male eardrum data (open squares) are taken from Gridi-Pappet al.9(Fig. 2d). Error bars are ±1 s.e.m. Full size image Laser Doppler vibrometry The vibration velocity amplitude spectrum of female TM in O. tormota is shown in Figure 4 (five ears of three females; mean±s.e.m.). For comparison, the male's data of mean velocity amplitude of TM in response to sound were taken from Gridi-Papp et al . [9] ( Fig. 2d ). The laser Doppler vibrometer measurements in females at 80 dB SPL revealed a spectral range, spanning 1 to 10 kHz with a peak sensitivity at 5 kHz. Above 10 kHz, the velocity amplitude dropped off at ∼ 30–40 dB, largely matching both the AEP amplitude versus frequency and the threshold versus frequency relationships observed in females ( Fig. 2b,c , red curves). In contrast, the laser Doppler vibrometry for males showed a wideband spectral range from 2 to ∼ 35 kHz with a peak sensitivity at 7 kHz (ref. 9 ). Figure 4: Vibration velocity amplitude of the tympanic membrane of O. tormota in response to sound. Velocity amplitude spectrum of the female's TM (solid diamonds), showing a peak around 5 kHz. Measurements at frequency range 1–40 kHz and 80 dB sound pressure level were made from five eardrums of three females. The male eardrum data (open squares) are taken from Gridi-Papp et al . [9] ( Fig. 2d ). Error bars are ±1 s.e.m. Full size image The results of behavioural experiments with gravid females, using the entire spectrum of male calls or only ultrasonic components, support our hypothesis that female O . tormota , unlike males, are insensitive to ultrasound. Electrophysiological recordings of AEPs and single TS units from the auditory brain further indicate that the upper frequency limit of the female is at ∼ 16 kHz, rather than at 20 kHz. Thus, there are remarkable differences in the auditory frequency sensitivity between the sexes in O . tormota . Female courtship call playback tests with males, performed indoors and in the field, show that receptive males perform perfect phonotactic movements and vocalization [2] . In this study, performed indoors, the playback of male calls also elicits considerable phonotactic movements and vocalization from gravid females. Data analysis indicates that the F 0 of the male's antiphonal calls range from ∼ 5 to 7 kHz (ref. 2 ), corresponding to the best frequency range (4–6 kHz) of the majority of auditory TS neurons in females ( Fig. 2c , red curve). The BEFs of most TS units in males are distributed from ∼ 6 to 10 kHz, a range comparable with the F 0 of the female calls ( ∼ 7.5–9.2 kHz) [2] . The higher-frequency-sensitive TS neurons in males are able to detect and tune to the female's courtship call, especially to the second harmonic (frequency range from ∼ 15 to 20 kHz; Fig. 1b ). Thus, in O . tormota the auditory-sensitive frequency in one sex correlates well with the F 0 of calls in opposite sex. The cross-matching of the auditory frequency sensitivity to the F 0 of vocalizations between the sexes of O. tormota allows frogs of one sex to more reliably perceive calls emitted by the opposite sex, thereby facilitating mate detection at night in a noisy habitat. This comprehensive data set is a confirmation of the matched-filter hypothesis (the receiver is matched to the sender's call spectrum) [10] . Nevertheless, a mismatch exists between the female auditory tuning ( Fig. 2c ) and the F 0 of the female calls ( ∼ 7.5–9.2 kHz; Fig. 1b ) in O. tormota , which is different from the findings for other frog species [11] . Why does not the females of O. tormota possess the capacity to detect ultrasound? Previous studies suggest that restricted hearing in frogs is largely due to the limited high-frequency response of their middle-ear ossicles [1] . The mechanical properties of the middle ear determine the frequency sensitivity of the amphibian auditory system [12] , while middle-ear size and ossicular mass in mammals limit the upper frequency of hearing [13] . Adult male and female O. tormota have sexually dimorphic middle ears. Males possess ear canals with a resonant frequency of ∼ 4.3 kHz, which may facilitate high-frequency hearing, and recessed tympana, which shortens and therefore reduces the mass of the middle-ear ossicles. Both low-mass ossicles and thin TMs facilitate transmission of high-frequency sounds to the inner ear [1] . Compared with the males, females have relatively large (a diameter of 3.4±0.1, versus 2.6±0.1 mm for males) and thicker (the thinnest part having a thickness of 30–40 μm, versus 3–4 μm in males) TMs, but no ear canal. The female TM velocity amplitude spectrum showed a distinct peak in sensitivity at frequencies around 5 kHz and a much reduced sensitivity above 10 kHz. Hence, both the inertia of the larger and thicker TMs and the heavy-mass ossicles (about 3 times heavier) in the females limits the upper frequency of hearing ( ∼ 16 kHz) to approximately half of the upper frequency limit in males ( ∼ 35 kHz). Similarly, sexual differences in the tympanic frequency responses were also observed in the American bullfrog ( Rana catesbeiana ) [14] , [15] . The middle ear of adult male bullfrogs showed a distinct peak in sensitivity at very low frequencies around 200 Hz that was entirely lacking in the female middle ear. Males and females did not differ in the frequencies at which they were most sensitive in the green treefrog ( Hyla cinerea ) [8] . It is worth noting that the larger TMs in female O. tormota were responsible for the lower auditory threshold of ∼ 10 dB compared with the males, this was also observed in two Hyla species [16] , where females also had lower basilar papilla thresholds. Previous work shows that the tonotopic organization of the cochlea has a crucial role in setting the frequency limits of cochlear sensitivity and hence in determining the bandwidth of hearing in mammals, birds and reptiles [17] . It is still not known whether the inner ear (including the hair cells, the basilar papilla and the tectorial membrane) in the concave-eared frogs has a significant role in the determination of the upper-frequency limit of hearing. Animals Female concave-eared frogs ( O. tormota ) were collected at night along Tau Hua Creek (30°06′ N, 118°10′ E) in Huangshan Hot Springs, China, in April and May of 2008–2010. Most gravid females were captured during amplexus and then released ( n =22) between 19:30 and 22:00 h, three females were captured while unamplexed. All females were kept individually in plastic baskets and maintained on a 12:12 h light–dark cycle. Behavioural experiments were conducted during the dark phase of the cycle in a quiet and darkened room, near to the frog's natural habitat. Electrophysiological recordings were made at the Institute of Biophysics (IBP), Beijing. Laser Doppler vibrometry was performed at Beihang University, Beijing. All experiments were conducted following the Animal Care and Use Guidelines approved by IBP, the Chinese Academy of Sciences. Behavioural experiments Females were brought into a quiet and darkened room, ∼ 1 km from the frog's natural habitat for phonotaxis tests with an ambient temperature and humidity at ∼ 22°C and ∼ 60%. The area (150 cm length×90 cm width) was padded with acoustic foams (thickness 50 mm; Charcoal-grey colour) and an isolated female frog was placed under a removable glass cover (inside diameter: 8.5 cm), 1 m in front of the loudspeakers. The three basic call-types of the male's vocalizations (long call, short call and staccato call) [2] , [4] and their filtered ultrasonic components were used as acoustic stimuli. The WAV files of the stimuli were stored on the flash memory of the Play Unit and broadcast through a loudspeaker (Fostex FE87E; pass band 0.1–40 kHz) and an ultrasonic loudspeaker (Polaroid; pass band 22–120 kHz) at 90 dB SPL and a rate of one stimulus per 15 s. The EVRs and phonotaxis of females were recorded under infrared illumination using a digital audio recorder (Sound Devices model 722, Sound Devices; 16-bit resolution, a sampling rate of 96 kHz) with a 1/4″ wideband omni-directional microphone and a preamplifier (40 BE and 26 CB, G.R.A.S. Sound & Vibration; 4 Hz–100 kHz) mounted on a tripod and placed 10 cm from the loudspeakers and a video camera (SONY HDR-SR7). The trajectories for each female frog were obtained from the video recordings. The jump distance and azimuthal angle were measured and phonotaxis analyses were performed as described in the study by Shen [5] . Electrophysiological recordings Seventeen females and thirty males were used in the electrophysiological study. Frogs were anaesthetized by immersion in a 0.3% solution of tricaine methanesulfonate (MS222) and wrapped in cotton gauze. Incisions were made in the skin on the dorsal surface of the head, and a small hole was made in the skull above the TS. After surgery, animals were placed on a rubber platform inside a sound-proof and anechoic room, and immobilized during the recording session with periodic addition of 0.1% MS222. Tone bursts (50-ms duration, 5-ms rise and fall times, presented at a rate of 1 s −1 ) were generated by an RP2.1 Enhanced Real-time Processor (Tucker Davis Technologies (TDT) System 3), and played from a loudspeaker (FE87E, Fostex Japan) positioned 50 cm from the frog's contralateral eardrum. The SPLs of the stimulation system were measured with a condenser microphone (Brüel and Kjaer 4135) and a sound level metre (Brüel and Kjaer 2610). Glass microelectrodes (impedance 1–10 MΩ) were used to record AEPs (averaged over 20 trials) and single-unit activities from the TS in response to tone bursts at a frequency range of 1–35 kHz. Neural signals were amplified (RA4PA Preamp and RA16 Medusa Base, TDT), monitored visually and extracted using BrainWare software and stored on a hard drive and analysed off-line. The BEF and frequency-threshold curves of single units were determined, as described in the study by Feng et al . [1] Laser Doppler vibrometry Using a single-point Doppler laser vibrometer (Polytec OFV-3001), the vibration velocity of the TM of the frogs was measured in response to acoustic stimuli at an angle normal to the TM. The frog was anesthetized by immersion in a bath of 0.3% MS-222 for 5 min. A single retroreflective hemispheric glass bead (diameter 30–50 μm; 3 M, Scotchlite) was carefully placed in the centre of the TM with fine-tipped tweezers to increase its reflectivity and maximize measurement precision, as described in the study by Gridi-Papp et al . [9] A custom-made foam base (4 cm length×2.5 cm width×3 cm height) reaching from the vent to the pectoral girdle was used to support the frog during vibrometry. Acoustic stimuli and tone bursts (5-ms rise–fall time, 50 ms duration, frequency 1–40 kHz, a rate of 1 s −1 ) were generated by a function generator (DG3061A, Rigol) and played at a 80 dB SPL at the TM from a loudspeaker (1–40 kHz; FE87E, Fostex) positioned at 25 cm from the TM. Vibration velocity amplitude of the TM was recorded by a Multifunction Data Acquisition DAQ (USB-6251, NI USA) at a sample rate of 80 kHz. Morphology The male and female O. tormota show evident sexual dimorphism (mean±s.d. ): snout-to-vent length 32.6±1.3 mm in males ( n =8) versus 61.9±2.1 mm in females ( n =5); head width 9.7±0.3 mm in males versus 14.3±0.3 mm in females; body weight 3.2±0.3 g in males versus 16.8±2.5 g in females. The morphology of the eardrum was measured based on horizontal sections stained with haematoxylin–eosin (50 μm in thickness). The eardrum diameter was 2.6±0.1 mm in males versus 3.4±0.1 mm in females, and the thickness of eardrum at the rim was 3–4 μm in males versus 30–40 μm in females. The middle ear ossicles were removed from the anaesthetized frogs and weighed by an electronic balance (Sartorius BP211D; Readability 0.01 mg), weighing 0.1 mg in males versus 0.23 mg in females. Statistical analyses Results were expressed as mean±s.d., or mean±s.e.m. as shown in Figures 2b,c and 4 . Data analysis was performed using analysis of variances followed by F -tests or Student's t -tests where appropriate. Values of P <0.05 were considered as significant. Both the kurtosis (ku) and skewness (sk) of the two data sets shown in Figure 3 were measured using Microsoft Excel. How to cite this article: Shen, J.-X. et al . Ultrasonic frogs show extraordinary sex differences in auditory frequency sensitivity. Nat. Commun. 2:342 doi: 10.1038/ncomms1339 (2011).